An infectious bat-derived chimeric influenza virus harbouring the entry machinery of an influenza A virus In 2012, the complete genomic sequence of a new and potentially harmful influenza A-like virus from bats (H17N10) was identified. However, infectious influenza virus was neither isolated from infected bats nor reconstituted, impeding further characterization of this virus. Here we show the generation of an infectious chimeric virus containing six out of the eight bat virus genes, with the remaining two genes encoding the haemagglutinin and neuraminidase proteins of a prototypic influenza A virus. This engineered virus replicates well in a broad range of mammalian cell cultures, human primary airway epithelial cells and mice, but poorly in avian cells and chicken embryos without further adaptation. Importantly, the bat chimeric virus is unable to reassort with other influenza A viruses. Although our data do not exclude the possibility of zoonotic transmission of bat influenza viruses into the human population, they indicate that multiple barriers exist that makes this an unlikely event. Zoonotic transmissions of avian influenza A viruses pose a constant threat to humans and can result in severe disease and death as currently demonstrated by viruses of the H5N1 (ref. 1 ) and H7N9 subtypes [2] . Furthermore, influenza A viruses are known to cause devastating pandemics in the human population as exemplified by the 1918 ‘Spanish’ H1N1 pandemic with an estimated 50 million human deaths [3] . The ability of influenza A viruses to reassort their segmented genomes further facilitates the generation of pandemic viruses. Pigs in particular are known to represent a mixing vessel for genetic reassortment because of their high susceptibility for co-infections with different influenza A virus strains from various species [3] , [4] , [5] . Our knowledge about influenza virus diversity was recently challenged by the identification of complete genomic sequences of a new type of influenza virus, designated H17N10, from little yellow-shouldered fruit bats ( Sturnira lilium ) from Guatemala [6] . Phylogenetic analysis of the haemagglutinin (HA) segment revealed that H17 is closely related to the HAs of influenza A viruses [6] , although structural and functional studies have indicated that this protein lacks a typical sialic acid-binding pocket and receptor-binding properties [7] , [8] . Similarly surprising, N10 is only distantly related to neuraminidases (NA) of influenza A and B viruses, and lacks detectable sialidase activity [9] , [10] . Despite these differences, phylogenetic analysis of the segments coding for the three polymerase subunits PB2, PB1 and PA, the nucleoprotein NP, the matrix protein M1 and M2, the non-structural protein NS1 and the nuclear export protein NEP suggests a closer relationship to influenza A viruses than to influenza B viruses [6] . Reconstitution of the polymerase complex demonstrated that the replication machinery of H17N10 is fully functional in human cells [6] . Moreover, the N-terminal domain of bat PA exhibits a tertiary structure and endonuclease activity similar to other conventional influenza A viruses [11] . Recently, a second bat influenza virus, designated H18N10, was identified from flat-faced fruit bats ( Artibeus planirostris ) from Peru, suggesting a broader distribution and diversity of bat influenza viruses at least in Central and South America [12] . The recent finding of new influenza A virus-like subtype genomes in bats expands the reservoir of potentially dangerous zoonotic influenza A viruses. Bats are known hosts of several life-threatening pathogens including Ebola virus, Hendra virus, rabies virus, severe acute respiratory syndrome coronavirus (SARS-CoV) and Middle East respiratory syndrome coronavirus (MERS-CoV) [13] . It is then of upmost importance to assess the host spectrum, reassortment capacity and possible therapeutic interventions for bat influenza viruses. However, the lack of infectious bat influenza virus isolates has impeded such assessments [6] , [12] . Here, we sought to determine the zoonotic potential of these novel bat influenza viruses using functional approaches, including the genetic reconstruction of infectious recombinant viruses with bat influenza virus genes. We find that both the nucleoprotein NP and the polymerase subunit PB2 support the reconstitution of influenza A but not of influenza B virus polymerases in human cells. Functional compatibility is also observed in the formation of virus-like particles (VLPs) using HA and NA of the influenza A virus strain A/SC35M and all internal bat proteins. Based on these findings, we generate an infectious virus containing six out of the eight bat virus genes and two genes of the influenza A virus strain A/SC35M coding for H7 and N7. This virus replicates well in mammalian cells and mice, but not in avian cells or in embryonated chicken eggs without further adaptation. Despite the inability to reassort with other influenza A viruses, our data suggest that zoonotic transmission of bat influenza viruses into the human population cannot be excluded. Functional complementarities of internal H17N10 proteins Based on the phylogenetic relationship between the known bat influenza viruses and influenza A viruses [6] , [12] , we speculated that components of the replication machinery between these viruses might be compatible. We therefore reconstituted the viral ribonucleoprotein/polymerase complex of several influenza A viruses in human HEK293T cells and substituted single polymerase subunits or NP with the corresponding H17N10 components. Bat influenza virus NP, and to a certain degree PB2, supported the polymerase activity of the mouse-adapted A/SC35M (H7N7) influenza A virus [14] , whereas replacement of PB1 and PA was not tolerated ( Fig. 1a ). Vice versa, bat influenza virus polymerase activity did not change if NP was substituted by the corresponding protein from SC35M, highlighting the functional compatibility of NP between these two strains ( Supplementary Fig. 1A ). Bat NP also supported the polymerases of all other tested influenza A virus subtypes, including A/Brevig Mission/1/18 and A/WSN/33 (both H1N1), A/Panama/2007/99 (H3N2) and A/Thailand/KAN-1/2004 (H5N1; Fig. 1a , Supplementary Fig. 1B ). In sharp contrast, no functional compatibility of the polymerases and NP of influenza B viruses B/Yamagata/73 and B/Lee/40 with any corresponding protein from the bat influenza virus was observed ( Fig. 1b ), suggesting a closer relationship of the replication machinery of H17N10 with influenza A than with influenza B viruses. NP from the bat influenza virus also supported the formation of SC35M-specific VLPs containing viral ribonucleoproteins coding for green fluorescent protein (GFP; Fig. 1c ), further highlighting the functional compatibility of this nucleoprotein. 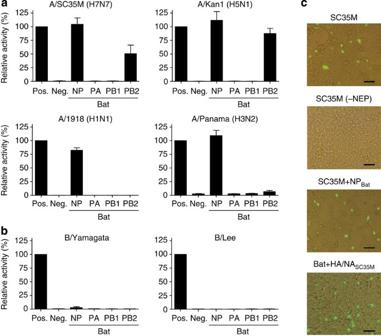Figure 1: Partial functional complementarities of H17N10 and influenza A virus internal proteins. (a,b) Relative polymerase activities for influenza A viruses (a) and influenza B viruses (b) were determined in HEK293T cells without (Pos.) or after substitution with the indicated single H17N10 components. Omission of the polymerase subunit PB1 (Neg.) served as a negative control. Shown are mean and standard deviation (s.d.) from three experiments. (c) Detection of virus-like particles containing viral ribonucleoproteins (vRNPs) with encapsidated reporter gene segment encoding GFP. Reconstitutions of virus-like particles were carried out with complete SC35M components PB2, PB1, PA, HA, NA, NP, M1, M2 and NEP (SC35M), omission of NEP (SC35M—NEP), substitution of SC35M NP with Bat H17N10 NP (SC35M+NPBat) or Bat PB2, PB1, PA, HA, NA, NP, M1, M2, NEP and HA and NA of SC35M (Bat+HA/NASC35M). Scale bar, 200 μm. Although we observed no GFP reporter signal if only bat virus components were used ( Supplementary Table 1 ), systematic exchange of bat and SC35M components revealed that infectious VLPs are efficiently formed with HA and NA of SC35M combined with the internal proteins of H17N10 ( Fig. 1c , Supplementary Table 1 ). Figure 1: Partial functional complementarities of H17N10 and influenza A virus internal proteins. ( a , b ) Relative polymerase activities for influenza A viruses ( a ) and influenza B viruses ( b ) were determined in HEK293T cells without (Pos.) or after substitution with the indicated single H17N10 components. Omission of the polymerase subunit PB1 (Neg.) served as a negative control. Shown are mean and standard deviation (s.d.) from three experiments. ( c ) Detection of virus-like particles containing viral ribonucleoproteins (vRNPs) with encapsidated reporter gene segment encoding GFP. Reconstitutions of virus-like particles were carried out with complete SC35M components PB2, PB1, PA, HA, NA, NP, M1, M2 and NEP (SC35M), omission of NEP (SC35M—NEP), substitution of SC35M NP with Bat H17N10 NP (SC35M+NP Bat ) or Bat PB2, PB1, PA, HA, NA, NP, M1, M2, NEP and HA and NA of SC35M (Bat+HA/NA SC35M ). Scale bar, 200 μm. Full size image Generation and characterization of chimeric bat influenza viruses Encouraged by these results, we attempted to generate reassortant viruses by reverse genetics [15] using authentic SC35M HA and NA segments and all other genomic segments from A/little yellow-shouldered bat/Guatemala/164/2009 (H17N10). However, no infectious viruses were obtained ( Fig. 2a ). To overcome potential packaging problems that might interfere with efficient virus production [16] , the coding regions of SC35M HA and NA were flanked with either the corresponding noncoding regions (NCR) of bat influenza virus (50-HA/NA SC35M ) or with an additional 97–114 nucleotides of the 5′ and 3′ end of the H17- and N10-coding regions (250-HA/NA SC35M ; Fig. 2a ). Successful rescue of infectious virus in human HEK293T cells and subsequent amplification in Madin-Darby canine kidney (MDCK) cells was only possible using the latter strategy ( Fig. 2a ). This is consistent with the presence of specific packaging signals at the 5′ and 3′ ends of the viral segments that include portions of the coding region, as it has been shown to be the case for conventional influenza A virus [16] . 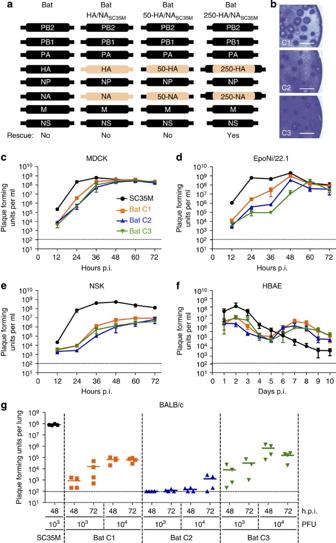Figure 2: Generation and growth of bat influenza virus harbouring the entry machinery of A/SC35M in mammalian cells and mice. (a) Cartoon depicting the segments of H17N10 or SC35M for rescue trials: all genomic segments of the H17N10 (Bat), the authentic SC35M HA and NA segments combined with the internal segments of H17N10 (Bat-HA/NASC35M), ORF of HA/NASC35Mwith the non-coding regions of H17N10 (Bat-50 HA/NASC35M) or ORF of HA/NASC35Mwith noncoding region and about 100 nt of the 5′ and 3′ coding sequences of H17N10 (Bat-250 HA/NASC35M). (b) Plaque phenotype of Bat C1, C2 and C3 on MDCK cells. Scale bar, 5 mm. (c–e) Viral growth of Bat C1, C2 and C3 in MDCK (canine), EpoNi/22.1 (bat) and NSK (swine) cells infected with an MOI of 0.01. Shown are mean and s.d. from three experiments. (f) Infection of primary human bronchial airway epithelial (HBAE) cells with 5 × 104PFU of the indicated viruses. Samples were obtained at the indicated days post infection and viral titres were determined by plaque assay. Error bars indicate s.d. of at least three to five experiments. (g) Viral lung titre (PFU per lung) in BALB/c mice (n=4/group) infected intranasally with the indicated amount of viruses after 48 or 72 h post infection (h.p.i.). The horizontal dotted line represents the detection limit (102PFU per ml). Figure 2: Generation and growth of bat influenza virus harbouring the entry machinery of A/SC35M in mammalian cells and mice. ( a ) Cartoon depicting the segments of H17N10 or SC35M for rescue trials: all genomic segments of the H17N10 (Bat), the authentic SC35M HA and NA segments combined with the internal segments of H17N10 (Bat-HA/NA SC35M ), ORF of HA/NA SC35M with the non-coding regions of H17N10 (Bat-50 HA/NA SC35M ) or ORF of HA/NA SC35M with noncoding region and about 100 nt of the 5′ and 3′ coding sequences of H17N10 (Bat-250 HA/NA SC35M ). ( b ) Plaque phenotype of Bat C1, C2 and C3 on MDCK cells. Scale bar, 5 mm. ( c – e ) Viral growth of Bat C1, C2 and C3 in MDCK (canine), EpoNi/22.1 (bat) and NSK (swine) cells infected with an MOI of 0.01. Shown are mean and s.d. from three experiments. ( f ) Infection of primary human bronchial airway epithelial (HBAE) cells with 5 × 10 4 PFU of the indicated viruses. Samples were obtained at the indicated days post infection and viral titres were determined by plaque assay. Error bars indicate s.d. of at least three to five experiments. ( g ) Viral lung titre (PFU per lung) in BALB/c mice ( n =4/group) infected intranasally with the indicated amount of viruses after 48 or 72 h post infection (h.p.i.). The horizontal dotted line represents the detection limit (10 2 PFU per ml). Full size image For further analysis, we plaque-purified three bat/SC35M chimeric viruses, designated Bat C1, Bat C2 and Bat C3, which differed in their plaque size in MDCK cells ( Fig. 2b ). Deep sequencing of the viral genomes revealed non-silent mutations in Bat C1 (NA V167I, PA S550R) and Bat C2 (PB1 E656G), respectively, whereas no mutation was found in the coding sequences of Bat C3 ( Supplementary Table 2 ) compared with published sequences [6] . All three plaque-purified viruses replicated to similar titres in MDCK cells of up to 10 8 plaque-forming unit (PFU) per ml ( Fig. 2c ). Efficient growth was also observed in the kidney-derived bat cell line EpoNi/22.1 ( Fig. 2d ), but not in the bat cell line CarperAEC.B-3 ( Supplementary Fig. 2A ). In newborn swine kidney (NSK) cells ( Fig. 2e ) and cells derived from newborn pig trachea (NPTr; Supplementary Fig. 2B ), all three viruses grew to similar titres of up to 10 7 PFU per ml. Viral replication was also evident in both human lung carcinoma epithelial cells (A549; Supplementary Fig. 2C ) and primary human bronchial airway epithelial (HBAE) cell cultures, although not to the same extent compared with SC35M ( Fig. 2f ). However, increased viral titres were observed in HBAE cells at later time points post infection (p.i. ; Fig. 2f ). Sequence analysis at day 7 p.i. excluded the acquisition of new adaptive mutations. Replication of Bat C3 in the bat cell lines EpoNi/22.1 and CarperAEC.B-3 was reduced at lower temperature (33 °C) and almost absent at 40 °C ( Supplementary Fig. 2D ). This suggests that the optimal temperature for viral growth of the bat/SC35M chimera is around 37 °C, consistent with the observation that the average temperature of Sturnira lilium is 36.4 °C (ref. 17 ), the bat species in which the H17N10 viral genomes were identified. Together, these data suggest that the bat influenza viral proteins in combination with HA and NA of SC35M fully support viral replication in various mammalian species, including primary HBAE cells, although, in general, the bat/SC35M chimeric viruses had showed slower replication kinetics and/or reached somewhat lower titres than the control SC35M virus in mammalian cells. To analyse the growth properties of bat/SC35M chimeric virus in vivo , BALB/c mice were intranasally infected with either 10 3 or 10 4 PFU of bat/SC35M chimeric viruses and lung titres were determined 48 and 72 h p.i., respectively. Bat C2 replicated poorly and reached, independent of the infection dose, maximal lung titres of 3 × 10 3 PFU per lung, whereas infection with Bat C1 and C3 resulted in higher lung titres of up to 10 6 PFU per lung ( Fig. 2g ). Viral titres of the latter two viruses remain elevated in lung and nasal turbinate 5–6 days p.i. ( Supplementary Fig. 3A and B). However, infection of BALB/c mice with up to 10 6 PFU of Bat C3 caused no weight loss and mortality ( Supplementary Fig. 3C ). Similar viral lung titres were observed 72 h p.i. in B6 mice infected with 10 4 PFU of Bat C1, C2 and C3 ( Supplementary Fig. 3D ). Intriguingly, poor replication of Bat C2 was also observed in B6 mice lacking an intact IFN response system (B6 mice devoid of STAT1; Supplementary Fig. 3D ), suggesting that the poor viral replication cannot be increased in the absence of a robust intact innate immune response. Chimeric bat viruses are poorly adapted to avian cells To study the growth properties of Bat C1, C2 and C3 in avian cells, chicken hepatocellular carcinoma epithelial (LMH) cells and chicken fibroblasts (DF-1) were infected at a multiplicity of infection (MOI) of 0.01. In LMH cells, growth of the chimeric viruses, especially of Bat C3, was severely compromised compared with SC35M ( Fig. 3a ). In contrast, all three viruses replicated in DF-1 cells to viral titres of up to 10 7 PFU per ml, although with slower kinetics than the SC35M control virus ( Fig. 3b ). 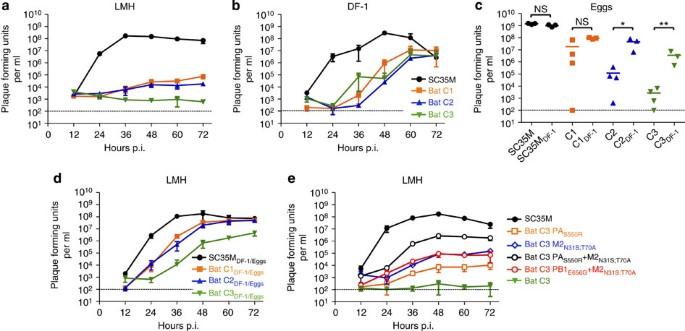Figure 3: Efficient viral growth in avian cells requires adaptation. (a,b) Viral growth of Bat C1, C2 and C3 in LMH and DF-1 cells infected with an MOI of 0.01. Note that viral replication in DF-1 cells was accompanied with mutations in the viral genome (Supplementary Table 4). Shown are mean and s.d. of three independent experiments. (c) Infection of embryonated eggs (n=3–4 per group) with 104PFU of MDCK-derived or DF-1-derived virus fromb. Student’st-test was performed to determine thePvalue. *P<0.05, **P<0.005, NS, not significant. (d) Infection of LMH cells with viruses passaged in DF-1 cells (b) and subsequently in eggs (c). (e) Infection of LMH cells with the indicated mutant viruses and SC35M. Horizontal dotted lines represent the detection limit. Shown are mean and s.d. of three independent experiments. Interestingly, all bat/SC35M reassortant viruses acquired several mutations during growth in DF-1 cells ( Supplementary Table 3 ). To test whether these mutations are involved in adaptation to avian cells, we compared the replication of DF-1 passaged viruses with the MDCK-derived viruses in embryonated chicken eggs using 10 4 PFU for either virus. Whereas the MDCK-derived Bat C2 and especially Bat C3 replicated only poorly in eggs, infection with Bat C1 resulted in high virus titres of up to 10 8 PFU per ml of allantoic fluid in some embryos ( Fig. 3c ). Following passaging MDCK-derived Bat C1 and Bat C2 viruses in embryonated eggs, analysis of virus quasispecies by deep sequencing identified several mutations, which resulted mainly in amino-acid changes in HA and PA ( Supplementary Table 4 ). Intriguingly, Bat C1, C2 and C3 that were passaged in DF-1 cells replicated to higher titres in embryonated chicken eggs than the corresponding viruses passaged in MDCK cells ( Fig. 3c ). The mutations acquired after one passage in DF-1 cells ( Supplementary Table 3 ) were also maintained in eggs ( Supplementary Table 4 ). Non-silent mutations resulted in amino-acid changes in HA, PA, M1 and most frequently in M2 (N31S; Supplementary Table 4 ). Following passage in embryonated chicken eggs, these viruses gained the ability to replicate more efficiently in LMH cells ( Fig. 3d ) than the original MDCK-derived viruses ( Fig. 3a ). These findings suggest that the mutations acquired in DF-1 cells and in ovo enhanced viral replication in avian cells. For further proof, we rescued Bat/SC35M chimeras (Bat-PA(S550R), Bat-M2(N31S,T70A), Bat-PA(S550R)M2(N31S,T70A) and Bat-PB1(E656G)M2(N31S,T70A), which contained the avian-like amino-acid mutations determined by deep sequencing ( Supplementary Tables 2 and 3 ). These viruses show enhanced viral growth in LMH cells compared with BAT C3, indicating that these avian-adapting mutations do indeed enhance viral replication in avian cells ( Fig. 3e ). To test whether the mutation in either PA (S550R) or PB1 (E656G) would increase the polymerase activity, we reconstituted the bat polymerase in either avian (LMH) or human cells (HEK293T) and compared the activity of these two mutant proteins with wild-type bat PA and PB1. As shown in Supplementary Fig. 4 , PA S550R as well as the PB1 E656G increased the polymerase activity in avian cells but not in human cells compared with wild-type bat polymerase. Together, these results indicate that the mutations observed following passage in DF-1 cells or chicken embryos led to increased replication in avian cells. Furthermore, this also suggests that bat influenza viruses are poorly adapted to avian hosts and adaptive mutations are required to overcome this species barrier. Figure 3: Efficient viral growth in avian cells requires adaptation. ( a , b ) Viral growth of Bat C1, C2 and C3 in LMH and DF-1 cells infected with an MOI of 0.01. Note that viral replication in DF-1 cells was accompanied with mutations in the viral genome ( Supplementary Table 4 ). Shown are mean and s.d. of three independent experiments. ( c ) Infection of embryonated eggs ( n =3–4 per group) with 10 4 PFU of MDCK-derived or DF-1-derived virus from b . Student’s t -test was performed to determine the P value. * P <0.05, ** P <0.005, NS, not significant. ( d ) Infection of LMH cells with viruses passaged in DF-1 cells ( b ) and subsequently in eggs ( c ). ( e ) Infection of LMH cells with the indicated mutant viruses and SC35M. Horizontal dotted lines represent the detection limit. Shown are mean and s.d. of three independent experiments. Full size image Bat chimeric viruses fail to reassort with influenza A viruses An important feature of influenza A viruses is the possibility to exchange genomic RNA segments with other influenza A viruses resulting in novel genotypes and phenotypes with zoonotic potential [3] , [4] , [5] , [18] . Importantly, attempts to generate H17N10 and SC35M reassortant viruses by reverse genetic approaches using authentic viral segments even with only a single bat genomic segment were unsuccessful ( Supplementary Table 5 ). Likewise, no reassortant viruses could be found after co-infection of MDCK cells with either Bat C3 and SC35M or Bat C3 and A/WSN/1933 (H1N1; Supplementary Table 6 ). This argues for incompatibilities of the H17N10 genomic RNA segments with segments of conventional influenza A viruses. In addition, the failure to generate a reassortant virus composed of authentic HA and NA segments of SC35M and the other six segments of H17N10 suggests RNA packaging incompatibilities ( Fig. 2a ). Bat chimeric viruses are resistant to amantadine treatment To evaluate options for therapeutic intervention against possible infections with bat influenza viruses, we tested several known antivirals. As expected, viral replication of chimeric viruses containing the N7 NA of SC35M was inhibited by the NA inhibitor zanamivir [19] ( Table 1 ). Similarly, efficient inhibition was also attained with the nucleoside analogue ribavirin [20] . However, all bat/SC35M chimeras were resistant to the M2 proton channel inhibitor amantadine [21] , consistent with the presence of a resistance-associated asparagine residue at position 31 (ref. 22 ); Supplementary Fig. 5 ). Accordingly, the egg-derived Bat C1 harbouring the N31S mutation ( Supplementary Table 4 ) was found to be highly sensitive to amantadine ( Table 1 ). Table 1 Determination of the 50% inhibitory concentration (IC 50 ) of amantadine, ribavarin and zanamivir on viral replication in MDCK cells by plaque-reduction assay. Full size table The reconstruction of a bat chimera influenza virus harbouring the entry machinery of an influenza A virus allowed us to prove that all genomic segments of A/little yellow-shouldered bat/Guatemala/164/2009 (H17N10), except for the HA and NA segments, encode functional gene products and support viral replication in mammalian cells and mice. Importantly, chimeric viruses could only be generated if the packaging elements of the two foreign RNA segments encoding HA and NA were replaced by the corresponding elements from the bat virus, suggesting that the packaging signals of the bat virus are not compatible with those of conventional influenza A viruses. Although the chimeric viruses replicated well in mammalian cells, viral replication was poor in avian cells and chicken embryos. This was rapidly overcome by the acquisition of mutations in various bat influenza virus gene segments, demonstrating the high plasticity of these gene products. In addition, this supports experimentally recent phylogenetic predictions of an independent evolution of bat influenza virus in bats without a history in avian species [23] . Despite partial functional complementarity of the internal components of H17N10 with those of a conventional influenza A virus, the envelope proteins of the bat virus seem to be strikingly different, as both H17 and H18 lack a sialic-acid-binding site [7] , [8] , [12] and N10 as well as N11 lack detectable NA activity [9] , [10] , [12] . This suggests that the cellular receptors for the bat influenza virus are different from those of conventional influenza A viruses. It is possible that bat influenza viruses make use of cellular receptors that are specific for certain bat species and/or tissues, which could explain why we did not succeed in generation of recombinant authentic bat H17N10 under laboratory conditions. M2, another component of the influenza A virus envelope, has an important role in the uncoating process of conventional influenza A viruses by facilitating the pH-dependent dissociation of M1 from NP [24] . Interestingly, in a VLP assay, the bat M2 protein was not functional in the context of the SC35M NP and M1 proteins, and vice versa SC35M M2 protein was not functional in the context of the bat virus NP and M1 proteins (see Supplementary Table 1 ). This indicates that the bat virus M2 protein does not cooperate with the NP and M1 proteins of SC35M. Although the chimeric virus with the homotypic bat virus NP, M1 and M2 proteins turned out to be resistant to amantadine, a mutant virus emerged during passage in avian cells, which was highly sensitive to this drug. This finding argues for a proton channel activity of the bat M2 protein. Whether this activity exhibits also a similar role in the viral life cycle as the conventional M2 proteins has to be further investigated. Although we cannot exclude zoonotic transmission of bat influenza virus, several barriers may exist that could prevent such events. Bat influenza viruses may bind to cellular receptors, which might be much more uncommon than sialic acids. In addition, the RNA packaging signals are different from those of conventional influenza A viruses thus impairing the emergence of reassortant viruses. Lack of reassortment with conventional influenza A viruses supports the inclusion of bat influenza viruses as a novel type (A-like) of influenza viruses. Moreover, M2 of the bat influenza virus did not functionally cooperate with NP and M1 proteins of conventional influenza A viruses. In addition, both PA and PB1 of H17N10 did not support polymerase activity of several influenza A virus polymerases. The probability that a non-human conventional influenza A virus infects people is already quite low, as even the most frequent human infections with non-human viruses are very low (39 human cases for H5N1 in 2013 and 375 human cases for H7N9 between May 2013 and February 2014 (WHO Global Influenza Program, http://www.who.int/influenza/en/ )). However, both H5N1 and H7N9 viruses are able to infect human cells, albeit with a different receptor specificity than human influenza viruses, and are able to reassort with human influenza viruses. The inability of bat-derived influenza viruses to infect human cells and to reassort with conventional influenza A viruses significantly reduces the risk of these viruses to cause human infections as compared with non-human conventional influenza viruses, such as H5N1 and H7N9. Given the enormous number of different bat species, the discovery of additional bat influenza viruses is likely. The more members of this fascinating new virus group will be detected the more we will be able to learn about their evolution and biology. In particular, research on the envelope glycoproteins HA, NA and M2 will reveal new aspects of influenza virus biology. Multiple alignment Protein sequences of M2 proteins of influenza isolates obtained from National Center for Biotechnology Information database were grouped according to their hosts resulting in data sets of 808 M2 protein sequences from swine, 1,329 sequences from avian, 840 sequences from human and 3 sequences from bat. The sequences were aligned within data sets using MUSCLE algorithm in Geneious software suite (v. 6.1.6; Biomatters). The four consensus sequences obtained from the alignments were compared using the consensus alignment tool calculating mean pairwise identities; the consensus was illustrated as sequence logo and transmembrane regions were predicted by TMHMM algorithm (all tools within Geneious software suite v. 6.1.6). Deep sequencing RNA from cell culture supernatants or embryonated eggs was extracted using QIAamp MinElute Virus Spin Kit (Qiagen) and further concentration and cleaning was done with Agencourt RNAClean XP magnetic beads (Beckman Coulter). RNA was quantified using Nanodrop UV spectrometer ND-1000 (Peqlab) and used as template for cDNA synthesis with cDNA Synthesis System (REF 11 117 831 001, Roche). Fragmentation of the cDNA applying a target size of 300 bp was done with Covaris M220 ultrasonicator. The sonicated cDNAs were used for library preparation using Illumina indices (Illumina) on a SPRI-TE library system (Beckman Coulter) using SPRIworks Fragment Library Cartridge II (for Roche FLX DNA sequencer; Beckman Coulter) without automatic size selection. Subsequently, upper and lower size exclusion of the library were done with Ampure XP magnetic beads (Beckman Coulter). The libraries were quality checked using High Sensitivity DNA Chips and reagents on a Bioanalyzer 2100 (Agilent Technologies) and quantized via quantitative PCR with Kapa Library Quantification Kit (Kapa Biosystems) on a Bio-Rad CFX96 Real-Time System (Bio-Rad Laboratories). Sequencing was done on an Illumina MiSeq using MiSeq reagent kit v3 (Illumina). Raw sequence data were analysed and mapped using the Genome Sequencer software suite (v. 2.8; Roche) and Geneious software suite (v. 6.1.6; Biomatters). Plasmid constructions pHW2000 rescue plasmids to generate SC35M have been previously described [25] . To generate the H17N10 rescue plasmids, the corresponding cDNAs of H17N10 (ref. 6 ), kindly provided by Ruben Donis (CDC), were amplified and cloned into pHW2000 vectors [15] . All sequences completely matched the previously published sequences [6] (GenBank accession numbers CY103880 , CY103881 , CY103882 , CY103883 , CY103884 , CY103885 , CY103886 , CY103887 and CY103888 ). The 50-HA, 50-NA, 250-HA and 250-NA pHW2000 vectors were generated by assembly PCR. In the 50-HA and 50-NA vector, the 3′ and 5′ NCR of the SC35M was replaced with the NCR of H17 and N10, respectively. For generation of the 250-HA pHW2000 rescue vector, the 3′ and 5′ NCR of the SC35M HA segments were replaced with nucleotides 1–131 and 1,621–1,782 of the bat HA sequence. For generation of the 250-NA pHW2000 rescue vector, the 3′ nd 5′ NCR of the SC35M HA segments were replaced with nucleotides 1–122 and 1,254–1,388 of the bat NA sequence. In addition, ATG codon in the coding sequence of the newly inserted Bat HA and NA ORFs were mutated to ACG to prevent initiation of translation at these sites. pCAGGS plasmids coding for bat (PB2, PB1, PA, HA, NP, NA, M2, M1, NEP) or SC35M [25] (HA, NA, M2, M1, NEP) influenza virus were generated by PCR amplification of the respective ORFs and subsequent ligated into suitable cloning sites. Cloned inserts coding for bat ORFs were verified by sequencing and were identical to the previously published sequences [6] . pCAGGS coding for SC35M PB2, PB1, PA and NP were described previously [25] . Plasmids to reconstitute the viral polymerase complexes of the various influenza A and B virus subtypes were described previously [26] , [27] , [28] , [29] . Cell lines Canine MDCKII (ref. 26 ), porcine NSK and NPTr cells [30] and human A549 (ref. 31 ) and HEK293T cells [32] were maintained in Dulbecco’s modified Eagle’s medium (DMEM) supplemented with 10% fetal calf serum (FCS), 2 mM L -glutamine, 100 U penicillin per ml and 100 μg streptomycin per ml. Chicken hepatocellular epithelial cell line (LMH) [33] and chicken fibrolast cells (DF-1) [34] were grown in DMEM supplemented with 8% (v/v) FCS, 2% (v/v) chicken serum, 2 mM L -glutamine, 100 U penicillin per ml and 100 μg streptomycin per ml. Bat cells EpoNi/22.1 (ref. 35 ) and CarperAEC.B-3 (ref. 36 ) were maintained in DMEM supplemented with 10% (v/v) FCS, 2 mM L -glutamine, 100 U penicillin per ml, 100 μg streptomycin per ml, 1 mM sodium pyruvate and 0.1 mM non-essential amino acids (NEAAs, Cyagen catalogue number NEAA-10201-100). Primary HBAE cells (MucilAir, Epithelix Sàrl) reconstituted in Transwells of 6.5 mm of diameter with a pore size of 0.4 μm (Costar 3470, Corning) were maintained in MucilAir Culture Medium. Infection of cell cultures and primary HBAE cells Transwells with approximately 5 × 10 5 cells were washed three times with pre-warmed (37 °C) phosphate-buffered saline (PBS) for 15 min and infected with 5 × 10 4 PFU of virus in 200 μl DMEM without serum for 1 h at 37 °C and washed with 200 μl MucilAir Culture Medium. To monitor viral replication efficiency, the apical surface was incubated with 200 μl of MucilAir Culture Medium for 30 min. Infectivity in the supernatant was determined by plaque assay in MDCKII cells. For infection of MDCKII, DF-1, NSK, NPTr, A549, LMH, EpoNi/22.1 or Carper AEC B-3 cells, cell cultures were washed with PBS and infected with viruses diluted in PBS with 0.2% bovine serum albumin (BSA). The infection solution was replaced 1 h p.i. by DMEM without serum and with 0.2% (v/w) BSA, 2 mM L -glutamine, 100 U penicillin per ml and 100 μg streptomycin per ml. Infection of embryonated eggs The indicated amount of viruses were applied to the allantoic sac and amniotic cavity of 9-day-old specific pathogen-free embryonated chicken eggs for 48 h at 37 °C. The allantoic fluid harbouring released viruses was collected. Infection of mice All animal experiments were performed in compliance with the German animal protection law (TierSchG). The state of Baden-Württemberg (Regierungspräsidum Freiburg) approved the animal experiments (reference number: 35-9185/G-13/110). BALB/c and B6 mice were obtained from Janvier, and B6- Mx1-STAT1 −/− mice (hereafter designated B6 STAT1 −/− mice) were kindly provided by Dr Staeheli. The latter mice were then bred locally. Six- to eight-week-old female mice were anaesthetized with a mixture of ketamine (100 μg per g body weight) and xylazine (5 μg per g body weight) administered intraperitoneally and inoculated intranasally with the indicated doses of viruses in 40 μl PBS containing 0.2% (v/w) BSA. Lung homogenates were prepared using the FastPrep24 system (MP Biomedicals). Briefly, after addition of 800 μl of PBS containing 0.2% (v/w) BSA, lungs were subjected to two rounds of mechanical treatment for 10 s each at 6.5 m s −1 . Tissue debris was removed by low-speed centrifugation. The LD 50 values were calculated based on the infectious dose (PFU). All animal work was conducted under BSL-3 conditions in accordance with the guidelines of the local animal care committee. Formation of VLPs VLPs were generated essentially as described [37] . Briefly, HEK 293T cells seeded in six-well plates were transfected with 1 μg of pCAGGS expression plasmid coding for PB2, PB1, HA, NA, NP and NEP, 0.1 μg of pCAGGS expression plasmid coding for PA and M2, and 2 μg of pCAGGS expression plasmid coding for M1, plus 1 μg of a GFP-encoding minigenome harbouring the A/WSN NCRs [38] , using the Lipofectamin transfection reagent (PAA Laboratories) in 2 ml of Opti-MEM (Invitrogen) according to the manufacturer’s protocol. Culture medium was replaced by DMEM containing 0.2% BSA 8 h post transfection. After 48 h, 1 ml of cell supernatant was transferred to MDCKII cells in six-well plates, infected with A/SC35M at an MOI of 5 and incubated for further 10 h. GFP signals were monitored by live imaging. Polymerase reconstitution assay For reconstitution of the polymerase complex in HEK293T or avian LMH cells [26] , pCAGGS plasmids (A/Brevig Mission/1/18, A/WSN/33, SC35M, A/Thailand/KAN-1/2004, B/Yamagata/73) [26] , [27] , [28] or pHW2000 plasmids (B/Lee/40, A/Panama/2007/1999) [29] encoding PB2, PB1, PA (each 50 ng) and NP (200 ng) were co-transfected with the firefly luciferase-encoding viral minigenome construct pPolI-FFLuc-RT (200 ng) and plasmid (pRL-SV40; 50 ng) coding for renilla luciferase. Expression of the minigenome, which is flanked by the NCRs of segment 8 of influenza A virus, is driven by the human or the avian polymerase I (ref. 26 ). Expression of renilla luciferase is under the control of the simian virus 40 promoter to normalize variations in transfection efficiency. Firefly and renilla luciferase activities were measured using the dual luciferase reporter assay 24 h post transfection [25] . Virus rescue The recombinant SC35M/bat chimeras were generated by the eight-plasmid reverse-genetics system as described previously [25] . The recombinant viruses Bat C1, C2 and C3 were plaque purified on MDCKII cells. Viral titres were determined by plaque assay on MDCKII cells. All work was conducted under BSL-3 conditions. Antiviral assay Amantadine, ribavirin and zanamivir were purchased from Sigma-Aldrich. Plaque reduction inhibition assay was carried out as described [39] with modifications. Briefly, confluent MDCKII cells were infected with 100 PFU per well of each virus in PBS with 0.2% (v/w) BSA for 1 h at 37 °C. After removal of the inoculums, cells were overlaid with DMEM containing 0.7% (v/w) low-melting point agarose supplemented with 0.2% (v/w) BSA, 2 mM L -glutamine, 5 mM sodium bicarbonate, 25 mM HEPES and antivirally active compounds zanamivir [19] , ribavirin [20] and amantadine [21] . These compounds were added at the following concentrations: zanamivir at 1.25, 12.5, 25, 50, 100 and 300 nM, ribavirin at 1.25, 12.5, 25, 50, 100 and 300 μM, and amantadine at 0.001, 0.01, 0.1, 1, 10 and 100 μM. After incubation for 48 h at 37 °C with 5% CO 2 , cells were fixed with formaldehyde and stained with crystal violet. Plaques were counted and standardized against the control with no drug. IC50 values were calculated using ED50plus v1.0 (Science Gateway). Virus reassortment assay and analysis To study reassortment events, MDCKII cells were co-infected with Bat C3 and SC35M, Bat C3 and WSN, or WSN and SC35M for 1 h at 37 °C with a MOI as indicated in Supplementary Table 6 . After removal of the media, cells were incubated for 40 s with 0.1 M glycine-HCl (pH 2.2) and subsequently maintained at 37 °C with 5% CO 2 in DMEM supplemented with 0.2% (v/w) BSA, 2 mM L -glutamine, 100 U penicillin per ml and 100 μg streptomycin per ml. After 48 h, virus-containing cell supernatants were collected and subjected to plaque assay on MDCKII cells. From each co-infection experiment, 100 plaques were picked and multiplied on MDCKII cells until cytophatic effect was visible, and cell culture (0.3 ml) supernatant was subjected to RNA purification. To establish the strain-specific reverse transcription PCR (RT–PCR) procedure, 30 individual plaques from each strain were picked and amplified. Viral RNA was obtained using QIAamp viral RNA Mini Kit (Qiagen) and eluted in 60 μl. Next, 5 μl of viral RNA were used as template to amplify influenza-specific cDNAs with a mixture of primers matching sequences in all eight segments from the three parental viruses ( Supplementary Table 7 ). The one-step reverse transcription (RT)-PCR consisted in a 1-h RT at 42 °C followed by 10 cycles of PCR, using Promega’s AccessQuick RT–PCR system (Promega). 5% of the resulting cDNA solutions were used as template in segment-specific real-time PCR using LightCycler 480 SYBR Green I Master. Primer pairs were chosen empirically to amplify fragments from the parental viruses with different melting temperatures. Single peak melting temperatures were used to identify the parental origin of each segment. In the case of six samples that yielded inconclusive results, viral supernatant of clones that were positive for Bat and SC35M was used to infect MDCK cells for further plaque purification of at least four clones. The viral segments of these individual plaque-purified clones were analysed by RT–PCR using strand-specific primer and partial sequencing. This revealed in all cases either Bat C3 or SC35M, indicating that a mixture of these two viruses, was present in the original six samples. How to cite this article: Juozapaitis, M. et al . An infectious bat-derived chimeric influenza virus harbouring the entry machinery of an influenza A virus. Nat. Commun. 5:4448 doi: 10.1038/ncomms5448 (2014).